Archaerhodopsin variants with enhanced voltage-sensitive fluorescence in mammalian andCaenorhabditis elegansneurons Probing the neural circuit dynamics underlying behaviour would benefit greatly from improved genetically encoded voltage indicators. The proton pump Archaerhodopsin-3 (Arch), an optogenetic tool commonly used for neuronal inhibition, has been shown to emit voltage-sensitive fluorescence. Here we report two Arch variants with enhanced radiance (Archers) that in response to 655 nm light have 3–5 times increased fluorescence and 55–99 times reduced photocurrents compared with Arch WT. The most fluorescent variant, Archer1, has 25–40% fluorescence change in response to action potentials while using 9 times lower light intensity compared with other Arch-based voltage sensors. Archer1 is capable of wavelength-specific functionality as a voltage sensor under red light and as an inhibitory actuator under green light. As a proof-of-concept for the application of Arch-based sensors in vivo , we show fluorescence voltage sensing in behaving Caenorhabditis elegans . Archer1’s characteristics contribute to the goal of all-optical detection and modulation of activity in neuronal networks in vivo . The study of brain circuitry encompasses three frames of reference: neuron-level spiking activity, circuit-level connectivity and systems-level behavioural output. A pervasive goal in neuroscience is the ability to examine all three frames concurrently. Fluorescent sensors, which enable measurements of simultaneous changes in activity of specific populations of neurons, are envisioned to provide a solution [1] , [2] , [3] , [4] , [5] . Successful detection of both high-frequency trains of action potentials and subthreshold events in neuronal populations in vivo requires a genetically encoded voltage indicator (GEVI) [6] with fast kinetics, high sensitivity and high baseline fluorescence. Recent developments of genetically encoded calcium [3] and voltage sensors [7] , [8] , [9] have yielded progress towards achieving this goal. The calcium sensor family GCaMP has been used to monitor populations of neurons in intact behaving organisms [4] . However, the detection of fast-spiking activity, subthreshold voltage changes and hyperpolarization is difficult with GCaMP due to its relatively slow kinetics and reliance on calcium, a secondary messenger, flux into the cell [3] , [10] , [11] . Newer iterations of voltage-sensitive fluorescent proteins based on fusions with circularly permuted GFP, for example, ASAP1 (ref. 7 ), improve on both the speed and sensitivity of previous sensors, for example, Arclight [12] , but are still limited by the ability to be combined with optogenetic actuators [13] , [14] , [15] . This spectral overlap prohibits the combined use of these sensors with opsins for all-optical electrophysiology. Currently available sensors are not able to meet all of the needs for optical imaging of activity in vivo , calling for continued efforts to evolve GEVIs. Archaerhodopsin-3 (Arch) [13] , [16] , a microbial rhodopsin proton pump that has recently been introduced as a fluorescent voltage sensor [17] , is fast and sensitive but suffers from low baseline fluorescence and strong inhibitory photocurrents. Previous optimizations of Arch successfully reduced photocurrents, for example, Arch D95N [17] and Arch EEQ [18] , and increased sensitivity and speed, for example, QuasArs [9] , but have still to enable its use in vivo . All previous in vivo voltage sensing has been accomplished using lower power of fluorescence excitation light than is possible with reported Arch variants to date [2] , [3] , [8] . For example, Arch WT [17] uses × 3,600 higher intensity illumination than ASAP1 (ref. 7 ). The high laser power used to excite Arch fluorescence causes significant autofluorescence in intact tissue [6] and limits its accessibility for widespread use. Here we report two Arch mutants (‘Archers’: Arch with enhanced radiance), Archer1 (D95E and T99C) and Archer2 (D95E, T99C and A225M) with improved properties for voltage sensing. These mutants exhibit high baseline fluorescence ( × 3–5 over Arch WT), large dynamic range of sensitivity (85% Δ F / F and 60% Δ F / F per 100 mV for Archer1 and Archer2, respectively) that is stable over long illumination times, and fast kinetics, when imaged at × 9 lower light intensity (880 mW mm −2 at 655 nm) than the most recently reported Arch variants [9] (and × 20.5 lower than Arch WT [17] ). We demonstrate that Archer1’s improved characteristics enable its use to monitor rapid changes in membrane voltage throughout a single neuron and throughout a population of neurons in vitro . Although Archer1 has minimal pumping at wavelengths used for fluorescence excitation (655 nm), it maintains strong proton pumping currents at lower wavelengths (560 nm). We show that this single protein, Archer1, is a bi-functional tool that provides both voltage sensing with red light and inhibitory capabilities with green light. Finally, we demonstrate that Archer1 is capable of detecting small voltage changes in response to sensory stimulus in the context of intact multicellular organisms such as C. elegans . The combination of D95E, T99C and A225M mutations was first identified in a site-saturation mutagenesis library of the proton pump Gloeobacter violaceus rhodopsin (GR) designed to evolve for spectral shifts [19] . Far-red shifted mutants of the GR library were then screened for fluorescence intensity in Escherichia coli , which revealed numerous hits with higher fluorescence than GR WT [19] . The corresponding mutations found in the most intensely fluorescent variants can be transferred to the homologous residues of Arch WT ( Supplementary Fig. 1 ) and greatly improve its quantum efficiency and absolute brightness [20] . The selected mutants were expressed in neurons to test if their improved characteristics were maintained in a mammalian system. Characterization of two new mutant Arch voltage sensors Arch variants designed with TS and ER export domains for enhanced membrane localization [21] ( Fig. 1a and Supplementary Fig. 1b ) were screened in neurons for enhanced baseline fluorescence and decreased photocurrents at imaging wavelengths, compared with Arch WT [17] . Of the Arch variants screened, Archer1 and Archer2 exhibited ~5 × and ~3 × increased fluorescence, respectively, over Arch WT ( Fig. 1a ). Archer1 and Archer2 also have × 55 and × 99 reduced photocurrents in response to 655 nm laser illumination, respectively, when compared with Arch WT ( Fig. 1b and Supplementary Fig. 2a ). Archer1 exhibits a peak current on initial laser exposure, which then reaches a residual average steady state of 5.6 pA, while Archer2 produces no peak current, and an average steady state of 3.1 pA ( Fig. 1b and Supplementary Fig. 2b,c ). Arch variants were also screened for increased voltage sensitivity and faster kinetics compared with previously reported variant Arch EEQ (ref. 18 ). Voltage sensitivity was measured as a fluorescence response to steps in membrane potential ranging from −100 mV to +50 mV. Due to Arch EEQ’s lower baseline fluorescence, its single-cell fluorescence traces show considerably more noise than those for Archer1 and Archer2 ( Fig. 1c ). Archer1 shows the highest voltage-sensitive fluorescence, as depicted by single-cell sensitivity measurements ( Fig. 1c and Supplementary Movie 1 ), and by the averaged traces ( Fig. 1d , Supplementary Fig. 3 ). Facilitated by Archer1’s increased baseline fluorescence, imaging can be done with short 1 ms exposure times and at lower laser intensities (880 mW mm −2 ) than previously published Arch-based sensors [9] , [17] , [18] . To characterize the stability of Archer1’s fluorescence, sensitivity was measured before and after prolonged laser illumination. Archer1 showed no reduction in voltage sensitivity over the 10–15 min timeframe measured ( Supplementary Fig. 4 ). 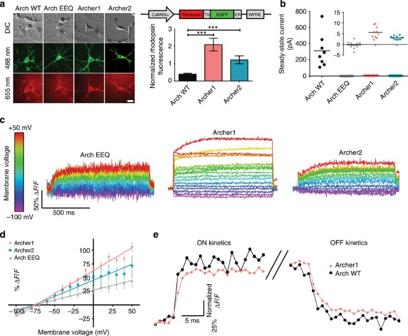Figure 1: Characterization of Arch variants in mammalian neurons. (a) Quantification of Archer1 (n=12) and Archer2 (n=11) fluorescence compared with Arch WT (n=13). Left—representative images of rhodopsin and fusion protein fluorescence; the published Arch EEQ–EYFP fusion18(Supplementary Table 1) is used, while all other sensors are fused to EGFP. Right graph—summary data. Baseline rhodopsin fluorescence normalized to EGFP fluorescence. Arch EEQ not included in comparison, as it has a different fluorescent protein fusion. Right construct—Arch-EGFP fusion vector design. Scale bar, 10 μm. (b) Average steady-state photocurrents generated by Arch WT (n=10) and different variants (n=9, 10 and 9 respectively for Arch EEQ, Archer1, and Archer2) in neurons voltage clamped atV=−50 mV. Inset shows low levels of photocurrents expanded to indicate differences between variants. (c) Fluorescent responses (imaged at 500 Hz) of single neurons expressing Arch EEQ, Archer1 and Archer2 to voltage-clamped steps in membrane potential. Neurons are held at −70 mV and stepped to voltages ranging from −100 mV to +50 mV in 10 mV increments. (d) Sensitivity of Arch variants measured as the functional dependence of fluorescence to change in voltage. Fluorescence changes are averaged over 1,000 ms voltage steps and plotted against voltage. Results exhibit linear dependence withR2values of 0.98, 0.95, and 0.99 for Archer1 (n=10), Archer2 (n=3) and Arch EEQ (n=5) respectively. (e) On/Off kinetics in response to a 100 mV step (−70 mV to +30 mV) for Archer1 (n=10) compared with Arch WT (n=6). %ΔF/Ffor each time point is normalized to the maximum step response (%ΔF/Faveraged over the whole step) (imaged at 1,000 Hz). Laser illumination for Arch WT, Archer1 and Archer2 (λ=655 nm;I=880 mW mm−2) is lower than that used for Arch EEQ (λ=655 nm;I=1,500 mW mm−2). Error bars represent s.e.m. ***P<0.001, NSP>0.05, unpaired student’st-test. Figure 1: Characterization of Arch variants in mammalian neurons. ( a ) Quantification of Archer1 ( n =12) and Archer2 ( n =11) fluorescence compared with Arch WT ( n =13). Left—representative images of rhodopsin and fusion protein fluorescence; the published Arch EEQ–EYFP fusion [18] ( Supplementary Table 1 ) is used, while all other sensors are fused to EGFP. Right graph—summary data. Baseline rhodopsin fluorescence normalized to EGFP fluorescence. Arch EEQ not included in comparison, as it has a different fluorescent protein fusion. Right construct—Arch-EGFP fusion vector design. Scale bar, 10 μm. ( b ) Average steady-state photocurrents generated by Arch WT ( n =10) and different variants ( n =9, 10 and 9 respectively for Arch EEQ, Archer1, and Archer2) in neurons voltage clamped at V =−50 mV. Inset shows low levels of photocurrents expanded to indicate differences between variants. ( c ) Fluorescent responses (imaged at 500 Hz) of single neurons expressing Arch EEQ, Archer1 and Archer2 to voltage-clamped steps in membrane potential. Neurons are held at −70 mV and stepped to voltages ranging from −100 mV to +50 mV in 10 mV increments. ( d ) Sensitivity of Arch variants measured as the functional dependence of fluorescence to change in voltage. Fluorescence changes are averaged over 1,000 ms voltage steps and plotted against voltage. Results exhibit linear dependence with R 2 values of 0.98, 0.95, and 0.99 for Archer1 ( n =10), Archer2 ( n =3) and Arch EEQ ( n =5) respectively. ( e ) On/Off kinetics in response to a 100 mV step (−70 mV to +30 mV) for Archer1 ( n =10) compared with Arch WT ( n =6). %Δ F / F for each time point is normalized to the maximum step response (%Δ F / F averaged over the whole step) (imaged at 1,000 Hz). Laser illumination for Arch WT, Archer1 and Archer2 ( λ =655 nm; I =880 mW mm −2 ) is lower than that used for Arch EEQ ( λ =655 nm; I =1,500 mW mm −2 ). Error bars represent s.e.m. *** P <0.001, NS P >0.05, unpaired student’s t -test. Full size image Sensitivity kinetics enables comparison across sensors The choice of a specific voltage sensor for a given experimental application depends on whether the sensor will yield a significant fluorescence change in response to a given voltage change within the timeframe of interest. Traditionally, sensitivity is quantified by measuring the steady-state fluorescence change for a step in voltage [7] , [8] , [9] , [12] , [17] , [18] , but the steady-state value does not provide information about the initial dynamics of the fluorescence response (sensor kinetics). The methods for kinetic analysis vary with different types of sensors. Following a previously used method for Arch-based sensor kinetics [8] , [18] , we compared Archer1 with Arch WT by normalizing the fluorescent responses of each sensor during a 1 s voltage step (−70 mV to +30 mV) to the steps maximum fluorescence. These results indicate very similar kinetics between the two ( Fig. 1e ), without addressing Archer1’s × 35 larger change in fluorescence. The large time scale of these voltage steps is not relevant for neuronal applications. However, normalizing over a shorter time scale produces variable results depending on the time point used for normalization ( Fig. 2b ). A method that takes into account the sensitivity of a sensor on the time scale relevant to an action potential is necessary. 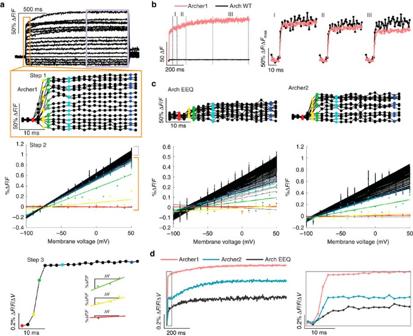Figure 2: A method for comparing different voltage sensors. (a) Overview of the method used to quantifySKi. Step 1: averaged fluorescence responses (imaged at 500 Hz) of neurons expressing Archer1 (n=10) to voltage-clamped steps in membrane potential. Neurons are held at −70 mV and then stepped to voltages ranging from −100 mV to +50 mV in increments of 10 mV. Step 2: voltage sensitivity of fluorescence is plotted for each time point and a linear fit is calculated. This step assumes a linear dependence of fluorescence on voltage. Step 3: the slope for each linear fit is plotted over time. This measure allows one to calculate %ΔF/Ffor a desired voltage change over any time scale. (b) Averaged change in fluorescence due to a 100 mV step (−70 mV to +30 mV) of Archer1 (n=10) compared with Arch WT (n=6) shows significant differences in response magnitude ( × 25–30). To compare the kinetics of the two sensors, normalization across the step is necessary. The maximum value within three different regions (I, II and III) is used as a normalization factor, resulting in different apparent kinetics and prompting the need for a different method for kinetic analysis. (c) Plotting the voltage sensitivity for each time point with linear best fits for Arch EEQ (n=5) and Archer2 (n=3) shows a slower rise to the steady-state value than Archer1 (n=10). (d) Summarizing theSKicomparison of Archer1, Arch EEQ and Archer2. Inset expands the first 40 ms. Laser illumination for Arch WT, Archer1 and Archer2 (λ=655 nm;I=880 mW mm−2) and for Arch EEQ (λ=655 nm;I=1,500 mW mm−2). Figure 2: A method for comparing different voltage sensors. ( a ) Overview of the method used to quantify SKi . Step 1: averaged fluorescence responses (imaged at 500 Hz) of neurons expressing Archer1 ( n =10) to voltage-clamped steps in membrane potential. Neurons are held at −70 mV and then stepped to voltages ranging from −100 mV to +50 mV in increments of 10 mV. Step 2: voltage sensitivity of fluorescence is plotted for each time point and a linear fit is calculated. This step assumes a linear dependence of fluorescence on voltage. Step 3: the slope for each linear fit is plotted over time. This measure allows one to calculate %Δ F / F for a desired voltage change over any time scale. ( b ) Averaged change in fluorescence due to a 100 mV step (−70 mV to +30 mV) of Archer1 ( n =10) compared with Arch WT ( n =6) shows significant differences in response magnitude ( × 25–30). To compare the kinetics of the two sensors, normalization across the step is necessary. The maximum value within three different regions (I, II and III) is used as a normalization factor, resulting in different apparent kinetics and prompting the need for a different method for kinetic analysis. ( c ) Plotting the voltage sensitivity for each time point with linear best fits for Arch EEQ ( n =5) and Archer2 ( n =3) shows a slower rise to the steady-state value than Archer1 ( n =10). ( d ) Summarizing the SKi comparison of Archer1, Arch EEQ and Archer2. Inset expands the first 40 ms. Laser illumination for Arch WT, Archer1 and Archer2 ( λ =655 nm; I =880 mW mm −2 ) and for Arch EEQ ( λ =655 nm; I =1,500 mW mm −2 ). Full size image Our proposed method for analysis, sensitivity kinetics ( SKi ), expands on the traditional method by providing %Δ F / F for any given voltage change over time ( Fig. 2a ). With this method, both the sensitivity and kinetics can be compared simultaneously among sensors. SKi is calculated by evaluating the slope of the fluorescence response to steps in voltage for each time point after the step’s initiation. The sensitivity slopes are then plotted over time ( Fig. 2a,c ). Characterization of the SKi for Arch variants reveals that Archer1 produces the largest changes in fluorescence of the sensors we tested ( Fig. 2d ), within any timeframe. Tracking action potentials in primary neuronal cultures Action potentials were evoked in cultured rat hippocampal neurons expressing Archer1 through current injection. Archer1 fluorescence is capable of tracking action potentials in both individual processes and the cell body ( Fig. 3a,b and Supplementary Movie 2 ). In addition, the magnitude and shape of dendritic fluorescence changes closely mimic that of the cell body in response to the same event. As predicted by the SKi , Archer1 fluorescence, with a >6 × increase in signal-to-noise ratio (SNR), more closely follows the electrical recording of action potentials than Arch EEQ at similar frequencies ( Fig. 3c,d ). Archer1 exhibits a large percentage change in fluorescence in response to action potentials (25–40% Δ F / F ), and can track 40 Hz firing rate as well as simulated changes in membrane voltage occurring at 100 and 150 Hz (>50% Δ F / F ) ( Fig. 3e,f ). The ability to follow action potential throughout neurons by imaging with significantly lower laser intensity (880 mW mm −2 ) is enabling for monitoring voltage-sensitive fluorescence in vivo . 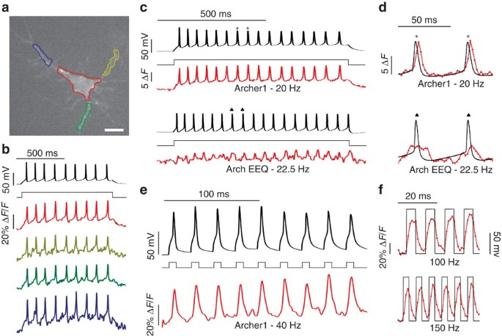Figure 3: Archer1 fluorescence tracks action potentials in cultured neurons. (a) Fluorescence of Archer1 expressing rat hippocampal neuron. Cell body and individual processes are outlined. Scale bar, 10 μm. (b) Fluorescence (imaged at 500 Hz) from single-trial optical and electrophysiological recordings of action potentials induced by a step current injection (800 ms, 50 pA) analysed for the color-matched somatic and dendritic areas outlined ina. (c) Fluorescence (imaged at 500 Hz) from single-trial recordings of action potentials in neurons expressing Archer1 and Arch EEQ. Firing of 20 and 22.5 Hz, respectively is generated through a step current injection (800 ms, 50 pA) in current-clamped cells. Fluorescence change is measured in absolute terms, as opposed to a percentage change, due to the lower baseline fluorescence of Arch EEQ. (d) Expanded regions of action potentials fromc. Archer1 shows ~2 × higher change in fluorescence and >6 × increase in SNR (24.03 versus 3.75) when compared with Arch EEQ, allowing it to better track action potential waveforms. Each fluorescent point is 2 ms apart. (e) Archer1 fluorescence (imaged at 1,000 Hz) successfully tracks action potentials in cultured rat hippocampal neurons at 40 Hz: higher limit for such cultures, generated through a succession of brief, large amplitude current pulses (5 ms, 500 pA). Individual action potentials at 40 Hz show ~40% change in ΔF/F. (f) Single-trial recording of high frequency (100 Hz and 150 Hz) voltage steps (−70 mV to +30 mV) are generated in neurons to test Archer1’s ability to detect fast trains of depolarization and hyperpolarization. Fluorescence changes (imaged at 1,000 Hz) exhibited by Archer1 are >50% ΔF/Ffor both frequencies and return near baseline between each pulse. Each fluorescent point is 1 ms apart. Laser illumination for Archer1 (λ=655 nm;I=880 mW mm−2) and Arch EEQ (λ=655 nm;I=1,500 mW mm−2). Fluorescence traces inb–ehave undergone background subtraction and Gaussian averaging. Figure 3: Archer1 fluorescence tracks action potentials in cultured neurons. ( a ) Fluorescence of Archer1 expressing rat hippocampal neuron. Cell body and individual processes are outlined. Scale bar, 10 μm. ( b ) Fluorescence (imaged at 500 Hz) from single-trial optical and electrophysiological recordings of action potentials induced by a step current injection (800 ms, 50 pA) analysed for the color-matched somatic and dendritic areas outlined in a . ( c ) Fluorescence (imaged at 500 Hz) from single-trial recordings of action potentials in neurons expressing Archer1 and Arch EEQ. Firing of 20 and 22.5 Hz, respectively is generated through a step current injection (800 ms, 50 pA) in current-clamped cells. Fluorescence change is measured in absolute terms, as opposed to a percentage change, due to the lower baseline fluorescence of Arch EEQ. ( d ) Expanded regions of action potentials from c . Archer1 shows ~2 × higher change in fluorescence and >6 × increase in SNR (24.03 versus 3.75) when compared with Arch EEQ, allowing it to better track action potential waveforms. Each fluorescent point is 2 ms apart. ( e ) Archer1 fluorescence (imaged at 1,000 Hz) successfully tracks action potentials in cultured rat hippocampal neurons at 40 Hz: higher limit for such cultures, generated through a succession of brief, large amplitude current pulses (5 ms, 500 pA). Individual action potentials at 40 Hz show ~40% change in Δ F / F . ( f ) Single-trial recording of high frequency (100 Hz and 150 Hz) voltage steps (−70 mV to +30 mV) are generated in neurons to test Archer1’s ability to detect fast trains of depolarization and hyperpolarization. Fluorescence changes (imaged at 1,000 Hz) exhibited by Archer1 are >50% Δ F / F for both frequencies and return near baseline between each pulse. Each fluorescent point is 1 ms apart. Laser illumination for Archer1 ( λ =655 nm; I =880 mW mm −2 ) and Arch EEQ ( λ =655 nm; I =1,500 mW mm −2 ). Fluorescence traces in b – e have undergone background subtraction and Gaussian averaging. Full size image Archer1 functions as a voltage sensor and inhibitory actuator All-optical electrophysiology requires an optical method for both sensing and perturbing cells. Recent work [9] presented a construct with dual capabilities: voltage sensing and neuronal activation at distinct wavelengths through co-expression of a sensor and a light-gated channel. Archer1 also provides two useful functionalities, both in a single protein. While minimally active with high intensity 655 nm laser illumination (880 mW mm −2 ), Archer1 is significantly more active at low intensity 560 nm light-emitting diode (LED) illumination (3 mW mm −2 ) ( × 51 at peak and × 35 at steady state) ( Fig. 4a,b ). The hyperpolarizing photocurrents generated by Archer1 in response to green light successfully inhibit action potentials, while red light does not ( Fig. 4c,d ). Thus, Archer1 is capable of inducing inhibitory currents with green light and sensing activity with red. 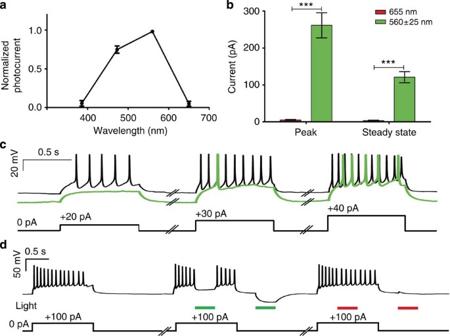Figure 4: Archer1 acts as either a sensor or actuator at separate wavelengths. (a) Normalized steady-state activation spectrum of Archer1 spanning wavelengths between 386–650 nm (n=11). (b) Currents induced by low intensity green LED illumination (n=8,λ=560±25 nm;I=3 mW mm−2) are significantly larger than those induced by high intensity red laser illumination (n=16,λ=655 nm;I=880 mW mm−2). (c) Archer1 exposed to green light successfully inhibits action potentials induced by step current injections (at 20, 30 and 40 pA) when compared with non-illuminated current injections in the same cell. (d) Action potentials induced by a 100 pA current injection (900 ms) are inhibited by a pulse of green light (300 ms;I=3 mW mm−2), while no inhibition of action potentials is observed with a pulse of red laser at the power used to excite fluorescence (300 ms;I=880 mW mm−2). In addition, with no current injection, hyperpolarization is observed with exposure to green, but not red light. Error bars represent s.e.m. ***P<0.0001, unpaired Student’st-test. Figure 4: Archer1 acts as either a sensor or actuator at separate wavelengths. ( a ) Normalized steady-state activation spectrum of Archer1 spanning wavelengths between 386–650 nm ( n =11). ( b ) Currents induced by low intensity green LED illumination ( n =8, λ =560±25 nm; I =3 mW mm −2 ) are significantly larger than those induced by high intensity red laser illumination ( n =16, λ =655 nm; I =880 mW mm −2 ). ( c ) Archer1 exposed to green light successfully inhibits action potentials induced by step current injections (at 20, 30 and 40 pA) when compared with non-illuminated current injections in the same cell. ( d ) Action potentials induced by a 100 pA current injection (900 ms) are inhibited by a pulse of green light (300 ms; I =3 mW mm −2 ), while no inhibition of action potentials is observed with a pulse of red laser at the power used to excite fluorescence (300 ms; I =880 mW mm −2 ). In addition, with no current injection, hyperpolarization is observed with exposure to green, but not red light. Error bars represent s.e.m. *** P <0.0001, unpaired Student’s t -test. Full size image Optical monitoring of cultured neuronal networks Fluorescent voltage sensors should enable the detection of spiking activity across all neurons in a population. Original Arch variants require the use of high optical magnification combined with binning and heavy pixel weighing [18] to detect modest changes in fluorescence, due to low baseline. Until recently [9] , these stringent imaging requirements had prevented microbial rhodopsin-based voltage sensors from being used to monitor multiple cells simultaneously. Archer1, similar to QuasAr [9] , by virtue of its increased fluorescence and higher SKi , allows simultaneous imaging of activity for a population of cells while perturbing only one of them through current injection ( Fig. 5a , schematic). Within the same optical field, we tracked the fluorescence of three cells with different behaviours: one showed a step change (due to an induced voltage step), one had spontaneous spikes that increased concurrently with the step and one remained unchanged ( Fig. 5a , traces). 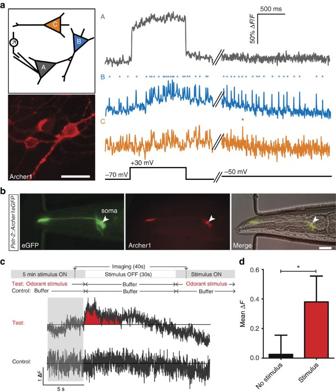Figure 5: Archer1 tracks activity in populations of cultured neurons and behaving worms. (a) Monitoring fluorescence in three Archer1 expressing cultured neurons with electrical stimulation of one cell. Cell A undergoes a voltage clamped 100 mV step and fluorescence changes in the population are measured simultaneously. Cell A exhibits a step-like increase in fluorescence corresponding to the voltage step. Cell B, whose fluorescence indicates spontaneous firing previous to the step, shows an increase in firing rate concurrent with the voltage step in Cell A, with continued firing after the step is completed. Fluorescence of Cell C appears not responsive to the voltage step in Cell A. Asterisks indicate action potential-like changes in fluorescence (~35–40% ΔF/Fincrease within 10 ms). Scale bar, 20 μm. (b)C. elegansexpressing Archer1 in one AWC neuron shows opsin fluorescence (λ=655 nm;I=880 mW mm−2, 100 ms exposure) co-localizing with fused EGFP fluorescence (λ=485±20 nm;I=0.05 mW mm−2, 100 ms exposure). Scale bar, 20 μm. (c) Top: behavioural paradigm: worms are stimulated with odorant (Isoamyl alcohol, IAA) for 5 min, flow is switched to buffer (S Basal) for 30 s, and then odorant flow is restored. On the same worm, a control is performed where odorant is replaced with buffer. Bottom traces: imaging of Archer1 fluorescence (250 Hz) is performed continuously for 40 s, starting 5 s before flow switch. Averaged ΔFtraces for two worms are shown. (d) Mean fluorescence of the 4-s time window after switch shows a significant increase with stimulus compared with no-stimulus controls (n=4 worms). Fluorescence traces imaged atλ=655 nm;I=880 mW mm−2. Fluorescence traces inaandbhave undergone background subtraction and Gaussian averaging. Error bars represent s.e.m. *P<0.05, paired student’st-test. Figure 5: Archer1 tracks activity in populations of cultured neurons and behaving worms. ( a ) Monitoring fluorescence in three Archer1 expressing cultured neurons with electrical stimulation of one cell. Cell A undergoes a voltage clamped 100 mV step and fluorescence changes in the population are measured simultaneously. Cell A exhibits a step-like increase in fluorescence corresponding to the voltage step. Cell B, whose fluorescence indicates spontaneous firing previous to the step, shows an increase in firing rate concurrent with the voltage step in Cell A, with continued firing after the step is completed. Fluorescence of Cell C appears not responsive to the voltage step in Cell A. Asterisks indicate action potential-like changes in fluorescence (~35–40% Δ F / F increase within 10 ms). Scale bar, 20 μm. ( b ) C. elegans expressing Archer1 in one AWC neuron shows opsin fluorescence ( λ =655 nm; I =880 mW mm −2 , 100 ms exposure) co-localizing with fused EGFP fluorescence ( λ =485±20 nm; I =0.05 mW mm −2 , 100 ms exposure). Scale bar, 20 μm. ( c ) Top: behavioural paradigm: worms are stimulated with odorant (Isoamyl alcohol, IAA) for 5 min, flow is switched to buffer (S Basal) for 30 s, and then odorant flow is restored. On the same worm, a control is performed where odorant is replaced with buffer. Bottom traces: imaging of Archer1 fluorescence (250 Hz) is performed continuously for 40 s, starting 5 s before flow switch. Averaged Δ F traces for two worms are shown. ( d ) Mean fluorescence of the 4-s time window after switch shows a significant increase with stimulus compared with no-stimulus controls ( n =4 worms). Fluorescence traces imaged at λ =655 nm; I =880 mW mm −2 . Fluorescence traces in a and b have undergone background subtraction and Gaussian averaging. Error bars represent s.e.m. * P <0.05, paired student’s t -test. Full size image Optical monitoring of sensory neurons in behaving C. elegans A major application for voltage sensors is all-optical neuronal activity monitoring in model organisms in which electrophysiological recordings are inherently difficult, for example, C. elegans. The aforementioned improved fluorescence and SKi of Archer1 have enabled us to extend its use from cultured cells to live, behaving nematodes. To test whether Archer1 will work in C. elegans , we examined the olfactory neuron AWC-ON (WormBase cell WBbt:0005832), one of the pair of C-type Amphid Wing cells. Previously, sensory-evoked Ca 2+ transients that were monitored using GCaMP show fluorescence increase on odour removal, which peaks within 10 s and gradually decreases over minutes post stimulation [22] . To monitor the small voltage changes underlying this effect, we expressed Archer1 in AWC-ON, and observed fluorescence changes in response to turning off the odorant stimulus (isoamyl alcohol) in anesthetized and non-anesthetized animals. According to Kato et al. [23] , the chemosensory responses in AWC neurons are not affected by the application of cholinergic agonist. As shown in Fig. 5b–d , Archer1’s fluorescence indicates that voltage transients peak within 2 s and end 10 s after turning off stimulus ( Fig. 5c and Supplementary Fig. 5 ). These observed fluorescence changes, which correspond to small reported changes in AWC membrane voltage [24] , validate the sensor’s in vivo utility. A combination of results from Archer1 and GCaMP experiments can be used to better understand the dynamics of C. elegans voltage-gated calcium channels. All-optical methods for in vivo recording will require a GEVI with fast kinetics, high sensitivity, high baseline fluorescence and compatibility with optical methods for controlling neuronal activity. Here we report an Arch mutant, Archer1, in which these combined improvements enable the accurate tracking of action potentials at high speed, the detection of simultaneous activity within populations of neurons, wavelength-specific inhibition of neuronal activity and the real-time observation of voltage changes in response to a stimulus in live nematodes. Fluorescence measurements of Archer1 and Archer2 were achieved at lower intensity of laser illumination than has been possible in experiments using previously reported Arch variants [9] , [17] , [18] . Reduction in excitation light intensity required for fluorescent measurements increases the accessibility of Arch-based voltage sensors and their potential use in vivo . Archer1 is an enhanced voltage sensor under red light and it also enables inhibition of action potentials under green light. Recent work has been done to generate an all-optical system for neuronal excitation and voltage sensing (Optopatch [9] ). Archer1, on the other hand, provides the first example of a combination of wavelength-specific sensing and hyperpolarization with a single protein. This wavelength-specific bi-functionality can enable all-optical dissection of a neural network through targeted inhibition and global fluorescence monitoring. Tools like Archer1 and Optopatch could be used for all-optical loss and gain of function circuit analysis, respectively. Voltage sensors can also provide insights into neuronal response to stimuli in organisms in which electrophysiology is challenging, such as Caenorhabditis elegans and Drosophila melanogaster . Archer1 represents the first genetically encoded voltage sensor that has been used in live, behaving nematodes. This work provides a foundation for more detailed characterization of cell types with unknown voltage dynamics as well as fast-spiking muscle cells in C. elegans [25] . Additional applications of this tool likely include other transparent organisms, such as, fly larvae and zebrafish, where a fluorescent voltage sensor could be used to dissect neural circuitry. Until recently, due to their low baseline fluorescence [6] , Arch-based sensors were not compatible with in vivo applications. This work on Archer1, as well as recent work on QuasArs [9] , demonstrates that Arch-based sensors are not fundamentally limited, but can be used for a variety of neuronal applications, including in vivo . Our data show that variants of Arch are capable of increased fluorescence, enabling practical detection, while retaining Arch WT's superior speed and dynamic range compared to XFP-based sensors [26] . Even though this work uses the lowest excitation intensity for an Arch-based sensor (<5% original illumination intensity of Arch WT [17] , ~60% of Arch EEQ [18] and 11% of QuasArs [9] ), it is still ~200 times higher than that for XFP-based sensors. Given the already fast kinetics and high sensitivity of Archer1, further enhancements to baseline fluorescence could result in a GEVI capable of detecting activity in mammalian neuronal populations in vivo . Ethics statement All experiments using animals in this study were approved by Institutional Animal Care and Use Committee (IACUC) at the California Institute of Technology. Sensor constructs Arch variant constructs were generated by first amplifying EGFP from FCK-Arch-GFP (Accession codes listed in Supplementary Table 1 ) and adding the ER export domain using GFPfwd_overlapTSend and FCK-GFPrev_ERexport primers ( Supplementary Table 2 ) to make EGFP-ER. Arch-TS was then amplified from pLenti-CaMKIIa-eArch3.0-EYFP ( Supplementary Table 1 ) using Archfwd and TSrev_into_GFPstart primers ( Supplementary Table 2 ), assembled with EGFP-ER using Archfwd and ERrev primers ( Supplementary Table 2 ), and subsequently cloned back into pLenti-CaMKIIa-eArch3.0-EYFP cut with BamHI and EcoRI restriction enzymes, to make pLenti-CaMKIIa-eArch3.0-EGFP. To make pLenti-CaMKIIa-Archer1-EGFP and pLenti-CaMKIIa-Archer2-EGFP, the D95E, T99C, and A225M mutations were introduced in the pLenti-CaMKIIa-eArch3.0-EGFP vector through overlap assembly PCR using Archfwd, ERrev, Arch3.0_D95E_T99C_fwd, Arch3.0_D95E_T99C_rev, Arch3.0_A225M_fwd, and Arch3.0_A225M_rev primers ( Supplementary Table 2 ) and subsequent cloning back into the backbone via BamHI and EcoRI sites. pLenti-Arch-EEQ ( Supplementary Table 1 ), an EYFP fusion, was used as a comparison. To make Pstr-2::Archer1eGFP::unc-54 3 ′ UTR , Archer1 was amplified from pLenti-CaMKIIa-Archer1-EGFP using Arch-NheI-AAA-F and Arch-EcoRI-R primers ( Supplementary Table 2 ) and inserted into the pSM vector using NheI and EcoRI sites. The C. elegans Kozak sequence AAA, and the restriction enzyme sites mentioned above were engineered into the primers [27] . The AWC-specific promoter, which is a 2 kb sequence 5′ to the start codon of str-2 , was amplified from genomic DNA using str-2p-SphI-F2(2K) and str-2p-AscI-R2 primers ( Supplementary Table 2 ) and cloned into the vector via SphI and AscI sites. Primary neuronal cultures Rat hippocampal cells were dissected from Wistar pups (postnatal days 0–1, Charles River Labs), and cultured at 37 °C, 5% CO 2 in Neurobasal media supplemented with B27, glutamine and 2.5% FBS. Three days after plating, glial growth was inhibited by addition of FUDR. Cells were transfected 4–5 days after plating with Arch WT and variants using calcium chloride. Neurons were imaged 3–5 days after transfection. Fluorescence imaging Imaging was performed concurrently with electrophysiology recordings of voltage- and current-clamped cultured rat hippocampal neurons. For both cultured neurons and in vivo C. elegans experiments, a Zeiss Axio Examiner.D1 microscope with a 20x 1.0 NA water immersion objective (Zeiss W Plan Apochromat × 20/1.0 DIC D =0.17 M27 75 mm) was used. A diode laser (MRL-III-FS-655-1.3W; CNI) with a 650/13 nm excitation filter, 685 nm dichroic mirror and 664 nm long-pass emission filter (all SEMROCK) was used for rhodopsin fluorescence excitation throughout. For cultured neuron experiments Arch WT, Archer1 and Archer2 fluorescence was excited with 880 mW mm −2 illumination intensity at the specimen plane, while for Arch EEQ, 1,500 mW mm −2 illumination intensity was used. Higher illumination intensity was used for Arch EEQ compared with other Arch variants due to its lower baseline fluorescence with our imaging setup. For C. elegans experiments, 880 mW mm −2 illumination intensity was used to visualize Archer1 fluorescence. For all experiments, fused EGFP fluorescence was imaged with 485±25 nm LED light using a Lumencor SPECTRAX light engine with quad band 387/485/559/649 nm excitation filter, quad band 410/504/582/669 nm dichroic mirror and quad band 440/521/607/700 nm emission filter (all SEMROCK) at 0.05 mW mm −2 . All fluorescence traces were recorded using an Andor Neo 5.5 sCMOS camera cooled to −30 °C at 500 or 1,000 Hz. Pixels were binned up to 0.54 μm × 0.54 μm to achieve the image acquisition speeds. All recordings were taken using Andor’s Solis software. Electrophysiology Conventional whole-cell patch-clamp recordings were done in cultured rat hippocampal neurons at >2 days post transfection. Cells were continuously perfused with extracellular solution at room temperature (in mM: 140 NaCl, 5 KCl, 10 HEPES, 2 MgCl 2 , 2 CaCl 2 , 10 glucose; pH 7.35) while mounted on the microscope stage. Patch pipettes were fabricated from borosilicate capillary glass tubing (1B150-4; World Precision Instruments, Sarasota, FL) using a model P-2000 laser puller (Sutter Instruments) to resistances of 2–5 MΩ. Pipettes were filled with intracellular solution (in mM): 134 K gluconate, 5 EGTA, 10 HEPES, 2 MgCl 2 , 0.5 CaCl 2 , 3 ATP, 0.2 GTP. Whole-cell patch-clamp recordings were made using a Multiclamp 700B amplifier (Molecular Devices, Sunnyvale, CA), a Digidata 1440 digitizer (Molecular Devices), and a PC running pClamp (version 10.4) software (Molecular Devices) to generate current injection waveforms and to record voltage and current traces. Patch recordings were done simultaneously with imaging for measurements of voltage-sensitive fluorescence. For sensitivity measurements cells were recorded in voltage clamp with a holding potential of −70 mV for 0.5 s and then 1 s voltage steps were applied ranging from −100 mV to +50 mV in 10 mV increments. Action potentials were generated in current clamp by current injection in either a long step (10–200 pA; 0.8 s) or in short pulses (100–500 pA; 2–10 ms). Patch-clamp recordings were done with short light pulses to measure photocurrents. Photocurrents induced by the excitation wavelength used for voltage sensing were measured using a 655 nm laser at 880 mW mm −2 . Photocurrents induced by green light were measured using 560±25 nm LED at 3 mW mm −2 . Photocurrents were recorded from cells in voltage clamp held at −50 mV with 3–10 light pulse trains (0.5 s each pulse; 2 s apart). Voltage changes induced by 655 nm laser at 880 mW mm −2 were measured in a current clamp mode with three 0.5 s light pulses separated by 2 s and zero current injection. To test for inhibitory capabilities of Arch mutants, pulses (300 ms) of illumination with either red laser (655 nm at 880 mW mm −2 ) or green LED (560±25 nm at 3 mW mm −2 ) were applied to cells during a 900 ms train of induced action potentials (generated in current clamp by current injections from 30–100 pA). Action spectra measurements were performed for the following wavelengths: 386±23 nm, 438±24 nm, 485±20 nm, 513±17 nm, 560±25 nm and 650±13 nm with light intensity matched across all experiments at 0.08 mW mm −2 . Each light pulse was delivered for 0.6 s with 10 s breaks between light pulses. All wavelengths were produced using LED illumination from a SPECTRAX light engine (Lumencor). Cell health was monitored through holding current and input resistance. Microinjection and germ line transformation in C. elegans The transgenic line used in this work is PS6666 N2; syEx1328[Pstr-2(2k)::Archer1eGFP( 75 ng μl −1 ) ; Pofm-1::RFP( 25 ng μl −1 )]. Pstr-2::Archer1eGFP::unc-54 3 ′ UTR was co-injected with a Pofm-1::RFP marker into Bristol N2 using the method described by Melo, et al. [28] The two plasmids were diluted to the desired concentration in water to make a 5 μl injection mix. The injection mix was spun down at 14,000 r.p.m. for 15 min and transferred to a new tube before injection to prevent needle clogging. Late L4 hermaphrodites were transferred to a newly seeded plate and maintained at 22 °C 1 day before injection. The microinjection was performed the next morning when the worms had become young adults. Worms were glued on a 2% agarose pad and covered with Halocarbon Oil (Halocarbon Products Corporation, HC-700) before injection. A quantity of 0.8 μl of the injection mix was loaded into the injection needle. For generating this particular transgenic line, 32 hermaphrodites (P 0 S) were injected for both arms of the gonad. 27 F 1 were identified 3 days after injection based on Pofm-1::RFP expression in coelomocytes. Among them, five eventually became stable lines. The best line used in this study was determined by the highest transmission rate and the strongest expression level of Archer1eGFP. C. elegans in vivo stimulation experiments Late L4 transgenic worms were transferred to a plate seeded with the mixture of OP50 and all-trans-Retinal (ATR) (Sigma-Aldrich, USA), and maintained at 22 °C in the dark 18 h before imaging. The final concentration of ATR in the mixture was 100 μm (diluted from 100 mM stock: 100 mg ATR powder dissolved in 3.52 ml 100% ethanol) using fresh OP50. Five times higher concentration of ATR was previously used for wild-type Arch activity in worms [29] . The microfluidic device is adapted for in vivo imaging [30] , [31] . The PDMS chip contains four buffer inlets, one worm-loading channel and one suction channel connected to house vacuum. Two buffer inlets in the middle are the ‘buffer’ and the ‘stimulus’ channels, which are loaded with the default solution S Basal medium and 1:1,000 isoamyl alcohol (Sigma-Aldrich), respectively. S Basal medium containing 0.15% phenol red (Sigma-Aldrich) is loaded in the side channels for detecting the laminar flow. An ATR-fed worm was first transferred to an empty NGM plate and washed in a drop of S Basal. It was then loaded in the microfluidic chip, where its nose was presented with either the buffer or the stimulus streams. The switch between buffer and stimulus stream was accomplished by changing the flow pressure from the side channels, which was regulated via an external valve controlled using a LabView script (National Instruments). The worm was exposed to the stimulus stream for 5 min (stimulus on), to the buffer stream for 30 s (stimulus off) and to the stimulus stream again. For performing the control experiments on the same worm, the flow switch remained the same but the stimulus channel was loaded with S Basal. Imaging of Archer1 fluorescence began 5 s before stimulus was switched off and lasted for 40 s. For anesthetized experiments only, 0.1% levamisole (Sigma-Aldrich) was added to the worm-loading channel to minimize movement artifacts. Data analysis Unless otherwise noted, all fluorescence analysis was done with raw measurements of cell fluorescence background subtracted. Cells and background regions were selected manually in ImageJ and fluorescence measurements were recorded for each region of interest (ROI) and background fluorescence was subtracted from cell fluorescence. Sensitivity analysis was performed using background subtracted fluorescence recordings. Baseline fluorescence (mean fluorescence of the cell 20 ms before voltage step) and step fluorescence (fluorescence over whole 1 s voltage step) were used to generate %Δ F / F traces for each voltage step. The mean %Δ F / F over the entire 1 s step was calculated for each voltage step and then plotted (%Δ F / F versus voltage step). On and off kinetics analysis was performed on fluorescence traces in response to a 100 mV step (−70 mV to +30 mV). Percentage change in fluorescence %Δ F / F for each time point is normalized to the maximum step response (%Δ F / F averaged over the whole step). SKi analysis was performed using time-locked, average %Δ F / F traces (voltage steps ranging from −100 mV to 50 mV in 10 mV increments) for all cells. At each time point throughout a voltage step ( t =0 at time of voltage step trigger), %Δ F / F was plotted versus the respective voltage step. A linear best fit was then performed for the %Δ F / F versus voltage step for each time point. The slope of the best fit for each time point was then plotted over time (%Δ F / F /voltage step versus time). SNR analysis for action potentials tracked by Archer1 and Arch EEQ fluorescence was performed. SNR was computed as SNR =abs( s–n )/ σ , where s =peak fluorescence during action potential, n =average of preaction potential noise and σ =s.d. of the preaction potential noise [2] . Worm AWC cell and background regions were selected manually in ImageJ, fluorescence measurements were recorded for each ROI and background fluorescence was subtracted from cell fluorescence. The ROI for the fluorescent cell was drawn to contain the cell soma for all time points of the experiment. Δ F is reported instead of %Δ F / F due to low detected baseline fluorescence. Calculating %Δ F / F would result in amplified signal, as well as amplified noise. Worm movement analysis was performed on the worm fluorescence traces, which were first thresholded so that only the pixels above a certain threshold are considered pixels of the cell. The cell location was then determined by averaging coordinates of pixels above the set threshold for the first frame in the 10,000 frame experiment to get the coordinates at the centre of the cell. A 70 × 70 pixel region around the centre of the cell was then set as the ROI. The centre of the cell was corrected by again taking the averaging coordinates of pixels above the set threshold within the 70 × 70 pixel region to eliminate any influence of pixel noise within the full frame. The corrected cell centre ( x c,1 ; y c,1 ) was then calculated for every frame of the 10,000 frame experiment ( x c,1 − x c,10,000 ; y c,1 − y c,10,000 ). The x and y displacement ( x d ; y d ) were calculated for each frame as the difference from x c,1 and y c,1 . The x d and y d were then plotted over time. Statistical methods Paired and unpaired student’s t -tests were performed using GraphPad Prism (version 6.04 for Windows, GraphPad Software, San Diego California, USA, www.graphpad.com ). How to cite this article : Flytzanis, N. C. et al. Archaerhodopsin variants with enhanced voltage-sensitive fluorescence in mammalian and Caenorhabditis elegans neurons. Nat. Commun. 5:4894 doi: 10.1038/ncomms5894 (2014).